EphB3 suppresses non-small-cell lung cancer metastasis via a PP2A/RACK1/Akt signalling complex Eph receptors are implicated in regulating the malignant progression of cancer. Here we find that despite overexpression of EphB3 in human non-small-cell lung cancer, as reported previously, the expression of its cognate ligands, either ephrin-B1 or ephrin-B2, is significantly downregulated, leading to reduced tyrosine phosphorylation of EphB3. Forced activation of EphB3 kinase in EphB3-overexpressing non-small-cell lung cancer cells inhibits cell migratory capability in vitro as well as metastatic seeding in vivo . Furthermore, we identify a novel EphB3-binding protein, the receptor for activated C-kinase 1, which mediates the assembly of a ternary signal complex comprising protein phosphatase 2A, Akt and itself in response to EphB3 activation, leading to reduced Akt phosphorylation and subsequent inhibition of cell migration. Our study reveals a novel tumour-suppressive signalling pathway associated with kinase-activated EphB3 in non-small-cell lung cancer, and provides a potential therapeutic strategy by activating EphB3 signalling, thus inhibiting tumour metastasis. Lung cancer is the major cause of malignancy-related death worldwide, and its incidence is rising in many countries. Non-small-cell lung cancer (NSCLC) comprises ∼ 80% of all lung cancers, with a gloomy prognosis and median survivals of less than 1 year [1] . Occurrence of metastases in distant organs is the major cause of death for the vast majority of lung cancer patients. In many cases, distant metastases have already developed by the time of the diagnosis of the primary lung lesions [2] . Mechanisms of development of lung cancer as well as lung cancer-derived metastases have received intense investigation over the last several years, and receptor tyrosine kinases have emerged as important therapeutic targets [3] , [4] . The Eph receptors constitute the largest subfamily of receptor tyrosine kinase superfamily. Binding to cell surface-associated ephrin ligands on neighbouring cells to generate bidirectional signals is a distinctive feature of Eph family. Eph kinase has been implicated in an increasing number of physiological and pathological processes in different organ systems [5] . Also, their roles in tumourigenesis have attracted growing interest recently [6] , [7] . Aberrant expression of Eph receptors and/or ephrins has been documented in various types of cancer cells [8] , [9] . However, the role of Eph kinase in tumour development and progression has remained controversial and paradoxical. For example, EphA2 promotes tumour growth and metastasis of breast cancer cells [10] , while its activation by ephrin-A1 ligand prevents tumour formation in xenograft models [11] . EphA2 and EphB4 are the most extensively studied Eph receptors in a variety of cancers. The role of EphB3 in cancer development has remained elusive. Our recent study illuminated the tumour-promoting property of EphB3 in NSCLC [12] . Overexpression of EphB3 was found in NSCLC patients, and silencing of EphB3 in NSCLC cells suppressed in vivo tumour growth and metastasis. Moreover, these pro-oncogenic effects were kinase-independent as even the kinase-deficient EphB3 (EphB3-KD) could promote tumourigenesis in nude mice. However, in the present study, we found that the cognate ligands of EphB3, ephrin-B1 and ephrin-B2, were significantly downregulated in the same cohort of NSCLC samples. These data indicated that the ligand-induced activity of EphB3 might have the potential to exert a tumour-suppressive role in NSCLC. Ephrin-stimulated 'forward' signalling of Eph receptors depends on autophosphorylation of the receptor, as well as subsequent phosphorylation and/or docking of various downstream effector proteins. Identifying the molecules interacting with Eph kinase is essential for clarifying the signal-transduction network downstream of Eph receptors. In the present study, we identified a novel EphB3-interacting protein—receptor for activated C-kinase 1 (RACK1)—by yeast two-hybrid assay. As a scaffold protein, RACK1 functions by recruiting different signalling molecules to discrete cellular compartments via protein–protein interactions at its seven WD40 repeats, and it has been reported to participate in a variety of cellular events [13] , [14] , [15] . Accumulating evidence suggests that RACK1 is also involved in tumourigenesis. For example, overexpression of RACK1 inhibits colon cancer cell growth by suppressing Src activity at G1 and mitotic checkpoints [16] . In addition, RACK1 mediates the interaction between integrin β-chain and activated protein kinase C-ɛ to promote integrin-mediated glioma cell adhesion and migration [17] . Our study reported here has made several novel observations. First, we demonstrate that kinase activation of EphB3 inhibits NSCLC cell migration both in vitro and in vivo . Second, this retardation of migration relies on a RACK1-mediated assembly of a PP2A/RACK1/Akt signalling complex. Taken together, these findings not only improve our understanding of the role of EphB3 in NSCLC, but also provide a potential therapeutic strategy for this cancer. Tyrosine phosphorylation of EphB3 is reduced in human NSCLC To explore the ligand-dependent function of EphB3, we examined the expression pattern of EphB3 ligands, ephrin-B1 and ephrin-B2, by real-time PCR in paired clinical samples from 60 NSCLC patients. The expression levels of ephrin-B1 and ephrin-B2 were significantly decreased in 38 of 60 (63%, P =0.006, Fig. 1a ) and 46 of 60 (77%, P <0.001, Fig. 1b ) tumour samples, respectively, as compared with the matched normal compartments. 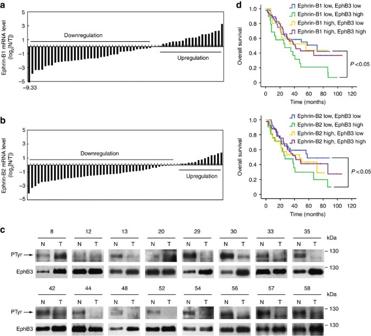Figure 1: Reduced tyrosine phosphorylation of EphB3 in paired NSCLC samples. (a,b) Quantitative real-time PCR results of relative expression level of ephrin-B1 (a) and ephrin-B2 (b) in 60 pairs of NSCLC and matched normal lung tissues. The expression of ephrin-B1 and ephrin-B2 were normalized to β-actin. (c) Tyrosine phosphorylation level of EphB3 in 16 pairs of random NSCLC samples. Tyrosine phosphorylation of the immunoprecipitated EphB3 was visualized with phosphotyrosine-specific antibody. T, tumour samples; N, matched normal tissues. (d) In total, 124 lung adenocarcinoma patients were classified into four groups according to their EphB3 and ephrin-B1 (upper) or ephrin-B2 (lower) expression levels as indicated in the figure. Kaplan–Meier method was applied to draw the curves. Statistical analyses were performed using Student'st-test. Figure 1: Reduced tyrosine phosphorylation of EphB3 in paired NSCLC samples. ( a,b ) Quantitative real-time PCR results of relative expression level of ephrin-B1 ( a ) and ephrin-B2 ( b ) in 60 pairs of NSCLC and matched normal lung tissues. The expression of ephrin-B1 and ephrin-B2 were normalized to β-actin. ( c ) Tyrosine phosphorylation level of EphB3 in 16 pairs of random NSCLC samples. Tyrosine phosphorylation of the immunoprecipitated EphB3 was visualized with phosphotyrosine-specific antibody. T, tumour samples; N, matched normal tissues. ( d ) In total, 124 lung adenocarcinoma patients were classified into four groups according to their EphB3 and ephrin-B1 (upper) or ephrin-B2 (lower) expression levels as indicated in the figure. Kaplan–Meier method was applied to draw the curves. Statistical analyses were performed using Student's t -test. Full size image Our previous studies showed that expression of EphB3 was dramatically upregulated in human NSCLC samples [12] . The inverse expression pattern between EphB3 receptor and its ligands in most tumour samples indicated that EphB3 may be hypophosphorylated in NSCLC, despite its high expression level. Thus, we examined the tyrosine phosphorylation level of EphB3 in 16 pairs of random samples. As expected, the tyrosine phosphorylation of EphB3 was significantly decreased in 75% (12/16) of tumour samples ( Fig. 1c ). Furthermore, evaluation of a published microarray data set of a cohort of 124 lung adenocarcinoma patients [18] revealed that high EphB3 expression combined with low ephrin-B1/B2 level was correlated with shorter overall survival ( Fig. 1d ). Taken together, these data indicate that phosphorylation of EphB3 may exert a suppressive effect on development and/or progression of the tumour. Ephrin-B1/B2–Fc treatment inhibits NSCLC cell migration To mimic the high expression level of EphB3 in human NSCLC, we overexpressed HA-tagged EphB3 in three NSCLC cell lines (H520, H23, A549), which expressed low levels of endogenous EphB3 ( Fig. 2a ). To investigate the ligand-induced function of EphB3, we purified both the extracellular domain of ephrin-B1 and ephrin-B2 by fusion to the Fc portion of mouse immunoglobulin-G (IgG). The addition of either ephrin-B1–Fc or ephrin-B2–Fc caused rapid phosphorylation of EphB3 in each of the EphB3-overexpressing NSCLC cell lines ( Fig. 2b ), associated with significant inhibition of serum-stimulated cell migration in Boyden chambers ( Fig. 2c ). However, no significant difference was found in cell proliferation and apoptosis on ligand treatment of these cells ( Supplementary Fig. S1a,b ). 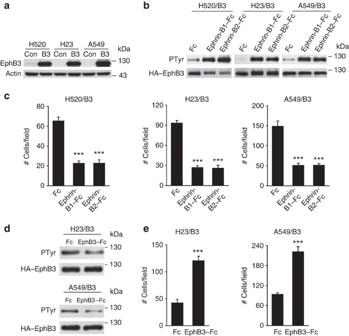Figure 2: EphB3 exhibits ligand-induced inhibition of NSCLC cell migration. (a) Ectopic overexpression of EphB3 in three NSCLC cell lines (H520, H23, A549, respectively). Cells were infected with lentivirus expressing either HA–EphB3 or vector control, followed by selection with puromycin for 3 days. Lysates were subjected to immunoblotting with anti-EphB3 and anti-β-actin (as a loading control). (b) HA–EphB3 immunoprecipitates using anti-HA from EphB3-overexpressing cells were probed with anti-phosphotyrosine antibody (pY100) and reprobed for anti-HA after ephrin-B1–Fc or ephrin-B2–Fc treatment. (c) EphB3-overexpressing cells were subjected to Boyden chamber cell migration assay with 10% fetal bovine serum in the lower chamber as chemoattractant, in the absence or presence of either ephrin-B1–Fc (2 μg ml−1) or ephrin-B2–Fc (2 μg ml−1). (d) HA–EphB3 were immunoprecipitated with anti-HA from EphB3-overexpressing cells, and the immunoprecipitates were probed with indicated antibodies after EphB3–Fc treatment. (e) EphB3 stable cells were subjected to Boyden chamber assay in the presence of Fc or EphB3–Fc (5 μg ml−1). For the quantification of Boyden chamber assay as incande, cell numbers from six random fields were counted. Numbers represent mean±s.d. Statistical significance was determined by Student'st-test. ***P<0.001 compared with Fc control–treated cells in each experiment. Figure 2: EphB3 exhibits ligand-induced inhibition of NSCLC cell migration. ( a ) Ectopic overexpression of EphB3 in three NSCLC cell lines (H520, H23, A549, respectively). Cells were infected with lentivirus expressing either HA–EphB3 or vector control, followed by selection with puromycin for 3 days. Lysates were subjected to immunoblotting with anti-EphB3 and anti-β-actin (as a loading control). ( b ) HA–EphB3 immunoprecipitates using anti-HA from EphB3-overexpressing cells were probed with anti-phosphotyrosine antibody (pY100) and reprobed for anti-HA after ephrin-B1–Fc or ephrin-B2–Fc treatment. ( c ) EphB3-overexpressing cells were subjected to Boyden chamber cell migration assay with 10% fetal bovine serum in the lower chamber as chemoattractant, in the absence or presence of either ephrin-B1–Fc (2 μg ml −1 ) or ephrin-B2–Fc (2 μg ml −1 ). ( d ) HA–EphB3 were immunoprecipitated with anti-HA from EphB3-overexpressing cells, and the immunoprecipitates were probed with indicated antibodies after EphB3–Fc treatment. ( e ) EphB3 stable cells were subjected to Boyden chamber assay in the presence of Fc or EphB3–Fc (5 μg ml −1 ). For the quantification of Boyden chamber assay as in c and e , cell numbers from six random fields were counted. Numbers represent mean±s.d. Statistical significance was determined by Student's t -test. *** P <0.001 compared with Fc control–treated cells in each experiment. Full size image In a reverse experiment, to disrupt the endogenous ephrin-B1/ephrin-B2–EphB3 interaction, we purified and tested the fusion protein composed of the extracellular domain of EphB3 and the Fc fragment of IgG. As we predicted, addition of EphB3–Fc to the EphB3-overexpressing H23 or A549 NSCLC cells reduced their EphB3 phosphorylation ( Fig. 2d ), and enhanced their serum-stimulated cell migration ( Fig. 2e ). Therefore, ephrin-B1/B2–EphB3 binding exerts a negative regulation on chemotactic cell migration. These experiments help to explain why there is a downregulation of ephrin ligands in NSCLC. Effects of distinct EphB3 kinase mutants on cell migration On the basis of previous studies on both EphB2 (refs 19 and 20 ) and EphB3 (ref. 21 ), two tyrosines (Y608 and Y614) in the juxtamembrane (JM) region of EphB3 are considered as the autophosphorylation sites, of which the unphosphorylated form forces the Eph kinase domain to interact with the JM region and keep the receptor in an autoinhibited state [5] . Substitution of both two tyrosine residues with glutamic acids relieves the autoinhibition and activates the kinase [20] , [22] . In contrast, replacement of these tyrosines with phenylalanines impairs the kinase activity [20] . Accordingly, to investigate the kinase-dependent function of EphB3, we constructed a haemagglutinin (HA)-tagged EphB3 kinase mutant that was constitutively active (EphB3-EE (Y608/614E)), a double-tyrosine-mutant (EphB3-FF (Y608/614F)), and a kinase-deficient EphB3 (EphB3-KD (K665R, ATP-binding site mutation)) [23] ( Fig. 3a ). 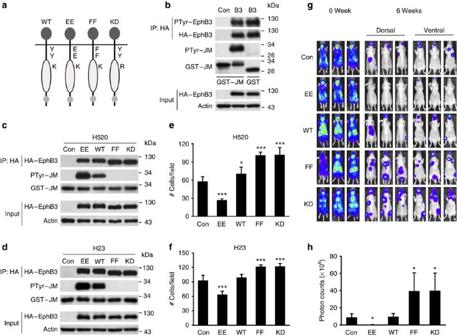Figure 3: Inhibition of cell migration andin vivometastatic seeding by EphB3 requires kinase activity. (a) Schematic models of different EphB3 kinase mutants used in the present study. WT, wild-type EphB3; EE, constitutively active EphB3, in which the two juxtamembrane tyrosines (Y608 and Y614) were replaced by two glutamic acid residues (E); FF, the two juxtamembrane tyrosines (Y608 and Y614) of EphB3 were replaced by two phenylalanine residues (F); KD, kinase-deficient EphB3, in which a lysine (K665) in the catalytic domain and responsible for ATP binding was mutated to a arginine residue (R). Both FF and KD mutations resulted in impaired kinase activity. (b) EphB3 kinase activity in immunoprecipitates from EphB3-transfected HEK 293T cells showing the specificity of the phosphorylation towards GST–JM, but not to GST alone. PTyr-GST–JM was detected with pY100 antibody. (c,d) HA-tagged EphB3 mutants or vector control were introduced into H520 (c) and H23 (d) cells via lentiviral infection. EphB3 kinase activity in each stable cell line was examined towards the exogenous substrate GST–JM. (e,f) Cell migratory ability between the stable cells in H520 (e) or H23 (f) was compared by Boyden chamber assay as described before. Numbers represent mean±s.d. from six random fields. *P<0.05, ***P<0.001 compared with vector-expressing control cells in each experiment. (g) Vector control, EphB3-WT- or EphB3 mutants-expressing H23 cells, all labelled with luciferase, were injected into the left ventricle of nude mice, and metastatic seeding was measured by luciferase activity. Images were obtained at week 0 and 6. (h) Mean photon counts of each group of mice (n=5) at 6 weeks were quantified and represented as the mean±s.d. *P<0.05, compared with control group of mice. The statistical differences were analysed by Student'st-test. Con, control; IP, immunoprecipitation. Figure 3: Inhibition of cell migration and in vivo metastatic seeding by EphB3 requires kinase activity. ( a ) Schematic models of different EphB3 kinase mutants used in the present study. WT, wild-type EphB3; EE, constitutively active EphB3, in which the two juxtamembrane tyrosines (Y608 and Y614) were replaced by two glutamic acid residues (E); FF, the two juxtamembrane tyrosines (Y608 and Y614) of EphB3 were replaced by two phenylalanine residues (F); KD, kinase-deficient EphB3, in which a lysine (K665) in the catalytic domain and responsible for ATP binding was mutated to a arginine residue (R). Both FF and KD mutations resulted in impaired kinase activity. ( b ) EphB3 kinase activity in immunoprecipitates from EphB3-transfected HEK 293T cells showing the specificity of the phosphorylation towards GST–JM, but not to GST alone. PTyr-GST–JM was detected with pY100 antibody. ( c , d ) HA-tagged EphB3 mutants or vector control were introduced into H520 ( c ) and H23 ( d ) cells via lentiviral infection. EphB3 kinase activity in each stable cell line was examined towards the exogenous substrate GST–JM. ( e , f ) Cell migratory ability between the stable cells in H520 ( e ) or H23 ( f ) was compared by Boyden chamber assay as described before. Numbers represent mean±s.d. from six random fields. * P <0.05, *** P <0.001 compared with vector-expressing control cells in each experiment. ( g ) Vector control, EphB3-WT- or EphB3 mutants-expressing H23 cells, all labelled with luciferase, were injected into the left ventricle of nude mice, and metastatic seeding was measured by luciferase activity. Images were obtained at week 0 and 6. ( h ) Mean photon counts of each group of mice ( n =5) at 6 weeks were quantified and represented as the mean±s.d. * P <0.05, compared with control group of mice. The statistical differences were analysed by Student's t -test. Con, control; IP, immunoprecipitation. Full size image To measure the kinase activity of these EphB3 mutants, we purified an in vitro substrate of EphB3: its own JM domain fused to glutathione- S -transferase (GST–JM). Immunoprecipitated EphB3 from EphB3-transfected HEK 293T cell lysate was able to phosphorylate the GST–JM substrate but not GST alone ( Fig. 3b ). Wild-type EphB3 (WT) and the kinase mutants were then introduced into H520 ( Fig. 3c ) and H23 ( Fig. 3d ) cells, and their in vitro kinase activities were assessed towards the GST–JM substrate, respectively. Cells expressing EphB3-EE mutant exhibited dramatically increased kinase activity compared with EphB3-WT-expressing cells, whereas few signals of phosphorylated GST–JM were detected with cells expressing either EphB3-FF or EphB3-KD. Chemotactic cell migration was examined in both H520 ( Fig. 3e ) and H23 ( Fig. 3f ) cells stably expressing EphB3-WT or one of the three EphB3 kinase mutants. Consistent with the result of ligand stimulation, the constitutively active EphB3-EE-expressing cells had significantly reduced cell migration ability, while EphB3-FF- and EphB3-KD-expressing cells showed enhanced migration capacity compared with either control or EphB3-WT-expressing cells. Effects of EphB3 kinase mutants on metastatic seeding in vivo To further examine the effects of these EphB3 kinase mutants in vivo , a bioluminescent murine model was used. H23 control, EphB3-WT and three mutant cell types were separately injected into the left ventricle of nude mice to induce experimental metastases. The metastatic seeding was measured by luciferase intensity. Consistent with the result of in vitro migration, EphB3-EE-expressing cells developed the fewest and smallest metastatic lesions. In contrast, EphB3-FF- and EphB3-KD-expressing cells had a greater capability to form more and larger metastatic foci, compared with control or EphB3-WT-expressing H23 cells ( Fig. 3g,h ). Taken together, EphB3 exerted a suppressive effect on both in vitro cell migratory capability and in vivo metastatic seeding in a kinase-dependent manner. RACK1 mediates Akt dephosphorylation by activation of EphB3 To elucidate the downstream signalling transduction of Eph receptors in tumour progression, we used yeast two-hybrid assay to screen EphB3-binding molecular partners, and identified RACK1 as a novel interactive protein. RACK1 is a scaffold protein that is able to interact simultaneously with several signalling molecules [24] . Both exogenous ( Fig. 4a ) and endogenous ( Fig. 4b ) coimmunoprecipitation and western blot assays confirmed the interaction between EphB3 and RACK1. Furthermore, binding of RACK1 to EphB3 positively correlated with the tyrosine phosphorylation level of the receptor ( Fig. 4c ), indicating that activation of EphB3 affected function of RACK1. As expected, silencing RACK1 desensitized EphB3-overexpressing H520 cells to the anti-migratory effects of ephrin-B1–Fc ( Fig. 4d ), suggesting that RACK1 was involved in the ligand-induced migratory inhibition exerted by EphB3. 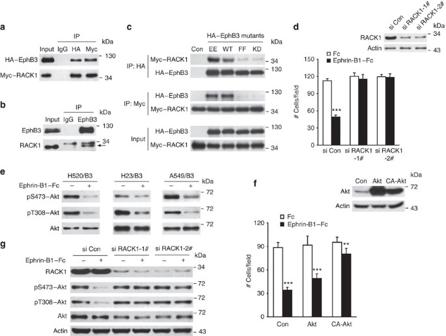Figure 4: Inhibition of cell migration by ephrin-B1–Fc treatment requires RACK1 adaptor function. (a) Exogenous association between RACK1 and EphB3. The plasmid encoding HA-tagged EphB3 was co-transfected with Myc-tagged RACK1 into HEK 293T cells. Immunoprecipitation (IP) was performed at 24 h after transfection with indicated antibodies. (b) Endogenous interaction between RACK1 and EphB3 in H520 cells. Immunoprecipitation was conducted using anti-EphB3, followed by immunoblotting with antibody against RACK1. (c) EphB3 kinase activity was essential for its interaction with RACK1. Vector control or indicated HA-tagged EphB3 mutants were co-transfected with Myc–RACK1 into HEK 293T cells. Immunoprecipitation was performed with either anti-HA or anti-Myc as indicated, 24 h after transfection. (d) Downregulation of RACK1 blocked ephrin-B1-Fc–induced cell migratory inhibition. RACK1 short hairpin RNA (shRNA) or scrambled control shRNA was introduced into EphB3-overexpressing H520 cells via lentiviral infection. Cell extracts were subjected to immunoblot to examine the knockdown efficiency. Chemotactic cell migration assay was performed as described before. Numbers represent mean±s.d. from six random fields. ***P<0.001 compared with Fc-treated si Con cells. (e) Ephrin-B1–Fc treatment induced S/T dephosphorylation of Akt. EphB3-overexpressing cells were stimulated with Fc (−) or ephrin-B1–Fc (+) for 15 min, total cell lysates were subjected to immunoblot with the indicated antibodies. (f) Constitutively active Akt (CA-Akt) rescued the migratory inhibition effect induced by ephrin-B1–Fc treatment. Vector control, Akt or CA-Akt was transiently transfected via FuGENE6 into H520/EphB3 cells. Transfected cells were subjected to Boyden chamber assay 24 h after transfection. Numbers represent mean±s.d. from six random fields. Statistical analyses were performed using Student'st-test. **P<0.01, ***P<0.001 compared with Fc-treated cells in each group. Immunoblot detected the expression levels of ectopic Akt and CA-Akt. (g) Silencing RACK1 in H520/EphB3 cells by short hairpin RNA abrogated ephrin-B1-Fc–induced Akt dephosphorylation. Figure 4: Inhibition of cell migration by ephrin-B1–Fc treatment requires RACK1 adaptor function. ( a ) Exogenous association between RACK1 and EphB3. The plasmid encoding HA-tagged EphB3 was co-transfected with Myc-tagged RACK1 into HEK 293T cells. Immunoprecipitation (IP) was performed at 24 h after transfection with indicated antibodies. ( b ) Endogenous interaction between RACK1 and EphB3 in H520 cells. Immunoprecipitation was conducted using anti-EphB3, followed by immunoblotting with antibody against RACK1. ( c ) EphB3 kinase activity was essential for its interaction with RACK1. Vector control or indicated HA-tagged EphB3 mutants were co-transfected with Myc–RACK1 into HEK 293T cells. Immunoprecipitation was performed with either anti-HA or anti-Myc as indicated, 24 h after transfection. ( d ) Downregulation of RACK1 blocked ephrin-B1-Fc–induced cell migratory inhibition. RACK1 short hairpin RNA (shRNA) or scrambled control shRNA was introduced into EphB3-overexpressing H520 cells via lentiviral infection. Cell extracts were subjected to immunoblot to examine the knockdown efficiency. Chemotactic cell migration assay was performed as described before. Numbers represent mean±s.d. from six random fields. *** P <0.001 compared with Fc-treated si Con cells. ( e ) Ephrin-B1–Fc treatment induced S/T dephosphorylation of Akt. EphB3-overexpressing cells were stimulated with Fc (−) or ephrin-B1–Fc (+) for 15 min, total cell lysates were subjected to immunoblot with the indicated antibodies. ( f ) Constitutively active Akt (CA-Akt) rescued the migratory inhibition effect induced by ephrin-B1–Fc treatment. Vector control, Akt or CA-Akt was transiently transfected via FuGENE6 into H520/EphB3 cells. Transfected cells were subjected to Boyden chamber assay 24 h after transfection. Numbers represent mean±s.d. from six random fields. Statistical analyses were performed using Student's t -test. ** P <0.01, *** P <0.001 compared with Fc-treated cells in each group. Immunoblot detected the expression levels of ectopic Akt and CA-Akt. ( g ) Silencing RACK1 in H520/EphB3 cells by short hairpin RNA abrogated ephrin-B1-Fc–induced Akt dephosphorylation. Full size image We further screened several signalling pathways to explore the downstream molecular mechanism mediating the ligand-dependent inhibition of chemotaxis by EphB3. We found that ephrin-B1–Fc treatment dramatically abrogated Akt phosphorylation at both the T308 and S473 sites ( Fig. 4e ). Furthermore, cells transfected with constitutively active Akt (T308D/S473D) became less sensitive to ephrin-B1-Fc–induced migratory suppression ( Fig. 4f ), indicating that decreased level of active Akt was responsible for the suppressive effect of ephrin-B1-Fc treatment on cell migration. Effects of Akt on cell proliferation and apoptosis during the experimental time period of chamber assay (6 h) were assessed, and no difference was observed ( Supplementary Fig. S2a,b ). Next, we explored whether the decreased level of Akt phosphorylation in response to ephrin-B1-Fc treatment was mediated by RACK1. As shown in Figure 4g , ephrin-B1-Fc stimulation had barely any effect on Akt phosphorylation in the RACK1 knockdown cells. In conclusion, the ligand-induced inhibition of cell migration by EphB3 was achieved by RACK1-mediated Akt dephosphorylation. PP2A is essential for ligand-induced Akt dephosphorylation Serine/threonine protein phosphatases have been reported to negatively regulate Akt activity in multiple cellular systems [25] . To test whether RACK1-mediated downregulation of Akt phosphorylation involves a protein phosphatase, we examined the effect of calyculin A (CA), a potent inhibitor targeting both PP1 and PP2A [26] , two very abundant phosphatases responsible for the dephosphorylation of many cellular proteins [27] , [28] . Pretreatment with CA completely blocked Akt dephosphorylation induced by ephrin-B1–Fc, even at a very low concentration ( Fig. 5a ). In addition, these experiments were repeated but this time using a more selective inhibitor okadaic acid (OA), which preferentially inhibits PP2A over PP1 within the concentration of 100 nM [29] . OA (100 nM) effectively antagonized Akt dephosphorylation responding to ephrin-B1–Fc stimulation ( Fig. 5b ), suggesting that PP2A was more likely involved in this event. 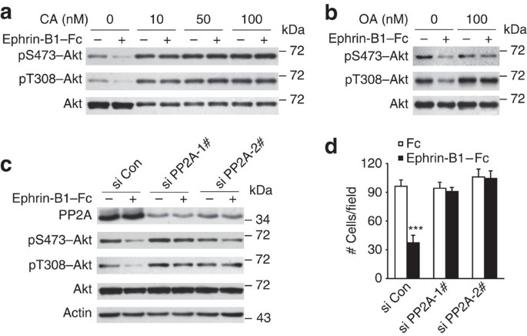Figure 5: PP2A phosphatase activity is required for ephrin-B1-Fc–induced Akt dephosphorylation and inhibition of cell migration. (a) Calyculin A (CA) prevented ephrin-B1-Fc–induced Akt dephosphorylation. H520/EphB3 cells were incubated for 30 min with the indicated concentrations of CA, followed by stimulation with 2 μg ml−1ephrin-B1–Fc or Fc control for 15 min. Lysates were probed with the indicated antibodies. (b) Okadaic acid (OA) prevented ephrin-B1-Fc–induced Akt dephosphorylation. H520/EphB3 cells were incubated for 4 h with OA at 100 nM, then stimulated and analysed as ina. (c) Akt dephosphorylation mediated by ephrin-B1–Fc was dependent on PP2A. H520/EphB3 cells were transfected with control short hairpin RNA (shRNA) or shRNA targeting PP2A catalytic subunit and stimulated with ephrin-B1–Fc or Fc as a control. Lysates were probed with the indicated antibodies. (d) Knockdown PP2A catalytic subunit in H520/EphB3 cells blocked ephrin-B1-Fc–induced cell migratory inhibition. Cell migration assay was performed as described before. Numbers represent mean±s.d. from six random fields. Statistical significance was determined by Student'st-test. ***P<0.001 compared with Fc-treated si con cells. Figure 5: PP2A phosphatase activity is required for ephrin-B1-Fc–induced Akt dephosphorylation and inhibition of cell migration. ( a ) Calyculin A (CA) prevented ephrin-B1-Fc–induced Akt dephosphorylation. H520/EphB3 cells were incubated for 30 min with the indicated concentrations of CA, followed by stimulation with 2 μg ml −1 ephrin-B1–Fc or Fc control for 15 min. Lysates were probed with the indicated antibodies. ( b ) Okadaic acid (OA) prevented ephrin-B1-Fc–induced Akt dephosphorylation. H520/EphB3 cells were incubated for 4 h with OA at 100 nM, then stimulated and analysed as in a . ( c ) Akt dephosphorylation mediated by ephrin-B1–Fc was dependent on PP2A. H520/EphB3 cells were transfected with control short hairpin RNA (shRNA) or shRNA targeting PP2A catalytic subunit and stimulated with ephrin-B1–Fc or Fc as a control. Lysates were probed with the indicated antibodies. ( d ) Knockdown PP2A catalytic subunit in H520/EphB3 cells blocked ephrin-B1-Fc–induced cell migratory inhibition. Cell migration assay was performed as described before. Numbers represent mean±s.d. from six random fields. Statistical significance was determined by Student's t -test. *** P <0.001 compared with Fc-treated si con cells. Full size image To further justify the involvement of PP2A, ephrin-B1-Fc–induced dephosphorylation of Akt was examined in both control cells and PP2A knockdown cells. As shown in Figure 5c , silencing PP2A resulted in reduced sensitivity of the cells to Akt dephosphorylation induced by ephrin-B1–Fc. Therefore, PP2A phosphatase was required for ephrin-B1-Fc–triggered Akt dephosphorylation, which was associated with EphB3 activation. Next, we assessed the role of PP2A in ephrin-B1-Fc–induced antimigratory effects. Knockdown of PP2A dramatically rescued the inhibitory migration induced by ephrin-B1–Fc ( Fig. 5d ). Taken together, these data indicate the critical importance of PP2A phosphatase activity in mediating Akt dephosphorylation and inhibiting cell migration subsequent to ligand activation of EphB3. Dynamic assembly of a PP2A/RACK1/Akt signalling complex To clarify further the interaction between RACK1, PP2A and Akt, we performed both exogenous ( Supplementary Fig. S3a ) and endogenous ( Fig. 6a ) coimmunoprecipitation experiments to verify the existence of a ternary PP2A/RACK1/Akt complex. Anti-RACK1 antibody precipitated endogenous PP2A, Akt, as well as the EphB3 receptor in both H520 and H23 cells ( Fig. 6a ), suggesting the interactions between these molecules. Next, we wondered whether the assembly of this complex was associated with the kinase activity of EphB3. 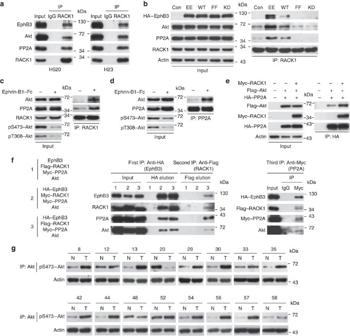Figure 6: Assembly of PP2A/RACK1/Akt signalling complex is regulated by ephrin-B1–Fc treatment. (a) RACK1 associated with endogenous PP2A, Akt and EphB3 in both H520 and H23 cells. Immunoprecipitation (IP) was performed with anti-RACK1, followed by immunoblotting with indicated antibodies. (b) HA–EphB3 mutants expressing H520 cells were subjected to coimmunoprecipitation assay with anti-RACK1, followed by immunoblotting for HA–EphB3, Akt and PP2A, respectively. (c,d) Increased interaction between RACK1 and either PP2A or Akt (c) or between PP2A and Akt (d) in the presence of ephrin-B1–Fc. H520/EphB3 cells were treated with Fc or ephrin-B1–Fc for 15 min, followed by immunoprecipitation with either anti-RACK1 (c) or anti-PP2A (d). (e) RACK1 enhanced interaction between PP2A and Akt. HA–PP2A was co-transfected with Flag–Akt into HEK 293T cells, either in the absence or presence of Myc–RACK1. Immunoprecipitation was performed with anti-HA, followed by immunoblotting with indicated antibodies. (f) Sequential coimmunoprecipitation to test for a complex formation of EphB3, RACK1, PP2A and Akt. HEK 293T cells were transfected with HA–EphB3 (or untagged EphB3 as control for the first immunoprecipitation), Flag–RACK1 (or Myc–RACK1 as control for the second immunoprecipitation), Myc–PP2A and Akt. The first step of immunoprecipitation was performed with anti-HA antibody. The complex was eluted by using HA peptide, followed by the second step of immunoprecipitation with anti-Flag. After 3× Flag peptide elution, the eluate was subjected to the final immunoprecipitation with anti-Myc or control mouse IgG. Protein samples from each step were then subjected to western blotting analysis separately by using indicated antibodies. (g) Phosphorylation levels of S473–Akt were assessed in the human NSCLC samples, which were examined for the level of pTyr-EphB3 inFigure 1c. Proteins were adjusted to equal amount according to the levels of β-actin in each pair of NSCLC tissues. Akt was immunoprecipitated with specific antibody, followed by immunoblotting for pS473–Akt. As shown in Figure 6b , levels of RACK1-interacted PP2A, Akt and EphB3 were remarkably increased in EphB3-EE-expressing cells, but significantly decreased in both EphB3-FF- and EphB3-KD-expressing cells, as compared with EphB3-WT-expressing cells. Consistently, western blot analysis of immunoprecipitates from EphB3-overexpressing H520 cells revealed a marked increase in the amount of PP2A and Akt precipitated with RACK1 ( Fig. 6c ), as well as an increased amount of Akt precipitated with PP2A ( Fig. 6d ) on ephrin-B1–Fc stimulation, suggesting the dynamic assembly of the PP2A/RACK1/Akt complex in response to EphB3 activation. To test whether RACK1 is an adaptor that bridges the interaction between PP2A and Akt, immunoprecipitation assays were carried out in HEK 293T cells. Co-transfection of RACK1 significantly increased the interaction between overexpressed PP2A and Akt ( Fig. 6e ), suggesting that RACK1 is a scaffolding intermediate for PP2A/Akt interaction. Furthermore, increased amounts of RACK1, PP2A and Akt were found in the immunoprecipitates of EphB3 complex upon ligand stimulation, revealing the recruitment of the PP2A/RACK1/Akt complex to kinase-activated EphB3 receptor ( Supplementary Fig. S3b ). Taken together, these data indicate that the PP2A/RACK1/Akt complex is assembled in response to EphB3 activation. Figure 6: Assembly of PP2A/RACK1/Akt signalling complex is regulated by ephrin-B1–Fc treatment. ( a ) RACK1 associated with endogenous PP2A, Akt and EphB3 in both H520 and H23 cells. Immunoprecipitation (IP) was performed with anti-RACK1, followed by immunoblotting with indicated antibodies. ( b ) HA–EphB3 mutants expressing H520 cells were subjected to coimmunoprecipitation assay with anti-RACK1, followed by immunoblotting for HA–EphB3, Akt and PP2A, respectively. ( c , d ) Increased interaction between RACK1 and either PP2A or Akt ( c ) or between PP2A and Akt ( d ) in the presence of ephrin-B1–Fc. H520/EphB3 cells were treated with Fc or ephrin-B1–Fc for 15 min, followed by immunoprecipitation with either anti-RACK1 ( c ) or anti-PP2A ( d ). ( e ) RACK1 enhanced interaction between PP2A and Akt. HA–PP2A was co-transfected with Flag–Akt into HEK 293T cells, either in the absence or presence of Myc–RACK1. Immunoprecipitation was performed with anti-HA, followed by immunoblotting with indicated antibodies. ( f ) Sequential coimmunoprecipitation to test for a complex formation of EphB3, RACK1, PP2A and Akt. HEK 293T cells were transfected with HA–EphB3 (or untagged EphB3 as control for the first immunoprecipitation), Flag–RACK1 (or Myc–RACK1 as control for the second immunoprecipitation), Myc–PP2A and Akt. The first step of immunoprecipitation was performed with anti-HA antibody. The complex was eluted by using HA peptide, followed by the second step of immunoprecipitation with anti-Flag. After 3× Flag peptide elution, the eluate was subjected to the final immunoprecipitation with anti-Myc or control mouse IgG. Protein samples from each step were then subjected to western blotting analysis separately by using indicated antibodies. ( g ) Phosphorylation levels of S473–Akt were assessed in the human NSCLC samples, which were examined for the level of pTyr-EphB3 in Figure 1c . Proteins were adjusted to equal amount according to the levels of β-actin in each pair of NSCLC tissues. Akt was immunoprecipitated with specific antibody, followed by immunoblotting for pS473–Akt. Full size image To determine whether RACK1, PP2A, Akt and EphB3 existed in one complex, we performed a sequential coimmunoprecipitation assay ( Fig. 6f ). HEK 293T cells were transfected with HA–EphB3, Flag–RACK1, Myc–PP2A and Akt. Anti-HA or anti-Flag antibody was used sequentially to pull down EphB3 or RACK1 complex, followed by elution with HA peptide or 3× Flag peptide, respectively. The final eluate was then immunoprecipitated with anti-Myc or control IgG, followed by western blotting to detect Akt. As shown in Figure 6f , Akt was present in the final immunoprecipitate but not in the control sample, indicating that EphB3, RACK1, PP2A and Akt were all in one complex. Akt is active in human NSCLC We have observed the reduced tyrosine phosphorylation of EphB3 in human NSCLC samples ( Fig. 1c ). We hypothesized that if activation of EphB3 kinase negatively regulated Akt activity in vitro , the phosphorylation level of Akt could be elevated in human NSCLC tissues. We then evaluated the p-Akt levels in the samples that we used to assess for pTyr–EphB3 levels ( Fig. 6g ). To exclude the detection of nonspecific signals, for each pair of NSCLC tissue as well as its matched normal lung tissue, Akt was immunoprecipitated from equal amount of tissue proteins, followed by western blotting for pS473–Akt detection. As shown in Figure 6g , phosphorylation levels of Akt were significantly increased in most (11/12) tumour samples that had decreased pTyr–EphB3 levels. Notably, in the tumour sample that had an elevated level of phospho-EphB3 (patient no. 20), Akt was dephosphorylated obviously. Taken together, these results lead us to propose that the cross-talk between EphB3 kinase and Akt signalling may contribute to malignant progression of NSCLC. In this study, we demonstrated the kinase-dependent suppressive function of EphB3 in NSCLC. Enforced phosphorylation of EphB3 by either ligand stimulation or genomic engineering resulted in inhibition of cell migration in vitro as well as metastatic seeding in vivo . Furthermore, we have identified a novel signalling pathway downstream of EphB3, which involved the formation of a protein complex comprising RACK1, PP2A and Akt in response to ligand stimulation ( Fig. 7 ). RACK1-mediated dephosphorylation of Akt by PP2A is responsible for ephrin-B1-Fc–induced inhibition of cell migration. 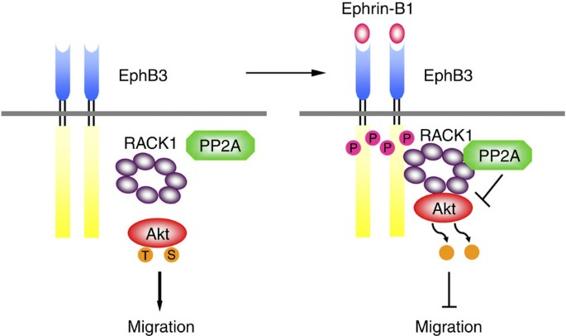Figure 7: Working model of the PP2A/RACK1/Akt signalling complex formed in response to EphB3 receptor activation in NSCLC cells. Ligand-dependent activation of EphB3 kinase results in PP2A and Akt recruiting to RACK1, which enhances the phosphatase/substrate interaction between PP2A and Akt, leading to Akt dephosphorylation and subsequent inhibition of cell migration. Figure 7: Working model of the PP2A/RACK1/Akt signalling complex formed in response to EphB3 receptor activation in NSCLC cells. Ligand-dependent activation of EphB3 kinase results in PP2A and Akt recruiting to RACK1, which enhances the phosphatase/substrate interaction between PP2A and Akt, leading to Akt dephosphorylation and subsequent inhibition of cell migration. Full size image Our recent work has identified the oncogenic roles of EphB3 that are independent of its kinase activity in NSCLC [12] . This study further demonstrates the kinase-dependent function of EphB3. In fact, the seemingly paradoxical function of Eph receptors in cancer has attracted increasing attentions in the past few years [30] , [31] , [32] . The pro- and anti-oncogenic properties exhibited by one Eph receptor appear to be regulated by the status of its cognate ligands. A typical example is the dual roles of EphB4 in breast cancer. Downregulation of EphB4 reduces breast cancer cell survival, proliferation as well as migration and invasion [33] . In contrast, ephrin-B2 stimulation of EphB4 inhibits cell proliferation, motility, invasion and tumour formation in vivo [34] . Similarly, while activation of EphA2 with its ligand ephrin-A1 inhibits chemotactic migration of glioma and prostate cancer cells, EphA2 overexpression promotes cell migration in a ligand-independent manner [31] . In this study, we find that EphB3 is overexpressed, but poorly tyrosine phosphorylated, in the primary samples of NSCLC, which may be ascribed to the decreased levels of both ephrin-B1 and ephrin-B2, indicating that the oncogenic effect of EphB3 is independent of ligand-induced kinase activation. Thus, cancer cells may circumvent the tumour-suppressive effect of Eph signalling by downregulating the expression of ephrin ligands, as an alternative to either losing Eph receptor expression or acquiring Eph receptor–inactivating mutations [35] , [36] . Further adding to the complexity of Eph receptor function in cancer cells, ephrin-B2-dependent EphB3/EphB4–Cdc42 signalling has been shown to enhance migration and cause defective contact inhibition of locomotion in prostate cancer [37] . Therefore, the tumour-promoting or tumour-suppressing effects of the Eph receptors appear to be determined on the cellular context. Most previous studies could not easily distinguish the contributions of Eph receptors specifically to metastasis regulation due to their mitogenic and/or antiapoptotic roles [34] , [38] . In contrast, our findings here show that ligand-stimulated EphB3 inhibits cell migration without exerting confounding influences on proliferation and apoptosis. Hence, inactivation of EphB3 by downregulating its ligands in the primary NSCLC may facilitate early development of metastatic disease. Statistical analysis revealed no correlation between ephrin-B1/ephrin-B2 expression and tumour stage, leading us to hypothesize that downregulation of EphB3 ligands may occur at a very early stage in the course of tumour development. Thereby, cells may be predisposed to a pro-metastatic behaviour at the onset of tumourigenesis, consistent with the highly metastatic potential of lung cancer. Investigation of the underlying signalling mechanisms is of great importance for developing effective therapeutic strategies. In this study, we have identified a novel EphB3-binding protein, RACK1, which has been previously reported to have multifaceted roles in various types of cancer. Here we showed that RACK1 recruited both PP2A and Akt in response to ephrin-B1-Fc–induced activation of EphB3, facilitating the phosphatase/substrate interaction by serving as a scaffold, and consequently abrogated Akt activity. Previous observations have shown that PP2A can interact with RACK1 in some circumstances [39] , [40] , [41] . For example, insulin-like growth factor 1 (IGF-1) controls the mutually exclusive association of RACK1 with PP2A and β1 integrin. IGF-1-mediated dissociation of PP2A from RACK1 results in decreased cellular PP2A activity, as well as increased cell migration [40] . Thus, RACK1 may regulate Akt activity by both enhancing the PP2A/Akt interaction and maintaining the phosphatase activity of PP2A. Besides, we also observed that the cell adhesion was suppressed when EphB3 kinase was activated. As mentioned above, the binding of RACK1 to integrin and PP2A are exclusive to each other. Therefore, on ephrin-B1 stimulation, the recruitment of PP2A by RACK1 may displace integrin, resulting in decreased cell adhesion. In addition, previous studies have implicated the role of RACK1 in regulating Akt activity in response to IGF-1 stimulatioin [42] , [43] , however, no interaction between RACK1 and Akt has been documented. Here we have demonstrated the dynamic association between these two molecules on ephrin-B1–Fc treatment. Taken together, RACK1 may participate in the regulation of Akt signalling through diverse mechanisms. In conclusion, we have shown the kinase-dependent tumour-suppressing effect of EphB3 on NSCLC cell migration as well as in vivo metastatic seeding, which is mediated by decreased Akt activity involving the formation of a ternary PP2A/RACK1/Akt complex. Our study unveils a novel signal mechanism downstream of Eph kinase in tumourigenesis, and suggests a potential EphB3-targeting therapeutic strategy for NSCLC that activates the kinase activity of the receptor to trigger its intrinsic tumour-suppressor functions. In fact, the suppressive effects of ligand stimulation have been implicated in the case of ephrin-B2/EphB4 cascade, as ephrin-B2–Fc treatment results in inhibition of breast cancer growth in nude mice [34] . Besides, specific antibodies to the extracellular domain of EphB3 could be taken into consideration, as monoclonal anti-EphA2 antibodies have been developed that can induce receptor phosphorylation and downregulation of EphA2 (ref. 44 ). Agonists similar to these are all attractive candidates for the new targeted therapy to inhibit malignant progression of NSCLC by stimulating EphB3 activation, thus abrogating pro-oncogenic effects of Akt phosphorylation. NSCLC tissue samples and cell lines Sixty pairs of primary NSCLC and their corresponding adjacent normal tissues, which were at least 5 cm away from the cancer, were obtained from NSCLC patients treated at Shanghai Chest Hospital (Shanghai, China), after their written informed consent. None of the patients received any radiochemotherapy. The fresh specimens were snap-frozen in liquid nitrogen and stored at −80°C until analysis. Our work was approved by the Institutional Review Board of the Institute for Nutritional Sciences (INS), Chinese Academy of Sciences (CAS). NSCLC cell lines H520 and H23 were purchased from Cell Bank of Type Culture Collection of Chinese Academy of Sciences, Shanghai Institute of Cell Biology, Chinese Academy of Sciences. NSCLC cell line A549 was a gift from Dr Jing Fang (INS, CAS). Antibodies and reagents Anti-EphB3 antibody (ab76885, 1:1,000) was purchased from Abcam (Cambridge Science Park, Cambridge, UK). Anti-β-actin (1:2,000) and anti-Myc (1:1,000) antibodies were obtained from Santa Cruz Biotechnology (Santa Cruz, CA, USA). Anti-RACK1 (1:2,500) and anti-PP2A catalytic (1:5,000) α-antibodies were from BD Transduction Laboratories (San Diego, CA, USA). Anti-HA (1:5,000), anti-Flag (1:5,000) antibodies and OA were from Sigma-Aldrich (Saint Louis, Missouri, USA). Phospho-tyrosine antibody pY100 (1:1,000), anti-Akt (1:1,000), anti-Akt (pS473) (1:1,000), anti-Akt (pT308) (1:1,000), horseradish peroxidase-conjugated secondary antibodies and CA were purchased from Cell Signaling Technology (Danvers, MA, USA). RNA preparation and real-time PCR Preparation of RNA and complementary DNA (cDNA) samples were performed as described earlier [45] . The primer pairs used for real-time PCR are listed in Supplementary Table S1 . The relative mRNA level of target genes to that of β-actin in clinical samples was calculated according to the methods described by Wang et al . [45] The statistical results were considered significant at P <0.05 and highly significant at P <0.01. All data analyses were carried out using SPSS 13.0 statistical software. Plasmid construction and transfection Full-length cDNA of EphB3 and EphB3-KD were subcloned from pBluescript, both of which were kindly provided by Dr Klaus Strebhardt (J W Goethe University, Germany), into pcDNA3-HA (kindly provided by Dr Xiang-jun Tong), respectively. EphB3 kinase mutants Y608/614E and Y608/614F were generated by site-directed mutagenesis of pcDNA3–HA–EphB3 by overlap extension of the target sites. The HA–EphB3-WT, -EE, -FF, -KD (together with the HA-tag) were then subcloned into pRDI-292 lentiviral expression vector and cells were selected with puromycin 3 days after virus infection. Plasmids encoding ephrin-B1–Fc, ephrin-B2–Fc or EphB3–Fc were kindly provided by Dr Hans-Christian Aasheim (Oslo University Hospital, Norway) for protein purification. PCMV–Myc–RACK1 and pCMV–HA–PP2A were gifts from Dr Yong Liu (INS, CAS). Flag–RACK1 and Myc–PP2A were generated by subcloning into pCMV–Tag2B and pCMV–Myc, respectively. Human Akt1 were subcloned from pcDNA3-Myr-HA-Akt1, purchased from Addgene, into pCMV-Tag2B with the FLAG tag in-frame at the N terminus. CA-Akt (T308D/S473D) was derived from pCMV–Tag2B–Akt1 with site-directed mutagenesis to introduce the desired mutations. Untagged EphB3 and Akt1 were subcloned into pcDNA3.1(−). Luciferase full-length cDNA was cloned into FG12 expressing construct and prepared for lentiviral expression. H23 cells were then labelled by luciferase lentivirus for in vivo metastasis assay. HEK 293T cells were transfected using the calcium phosphate precipitation method, and NSCLC cells were transfected using FuGENE6 Transfection Reagent (Roche Applied Sciences, Penzberg, Germany). Cell migration assay Chemotactic cell migration assay was performed using a 12-well Boyden chamber as described elsewhere [34] . Briefly, the underside of the filter was coated with 50 μg ml −1 rat tail collagen type I at 4°C overnight. Cells (5×10 4 ) in 1% fetal bovine serum were plated in the top of insert. Either ephrin-B1–Fc, ephrin-B2–Fc, EphB3–Fc or Fc was added to the lower chamber together with 10% fetal bovine serum. The chamber was then incubated at 37°C for 4–6 h. Cells that did not migrate through the pores of the filter were manually removed with a rubber swab. Cells that migrated to the underside of the filter were stained with eosin and photographed using an inverted microscope. In vivo metastatic seeding H23 cells were labelled with luciferase-expressing lentivirus before use. Cells (1×10 6 ) were injected into the left ventricle of 6-week-old nude mice (five mice for each group). The metastatic lesions were monitored by luciferase expression, which was determined by using luciferin (Xenogen, Alameda, CA, USA) and an in vivo imaging system (Xenogen). In vitro kinase assay GST–JM fusion protein was generated by subcloning a PCR product including the JM tyrosines of the human EphB3 (sequence CLRK ... DVSC) in frame with GST into the bacteria expression vector pGEX-4T-1. Protein was produced in BL21 bacteria and purified using a glutathione matrix column. For the in vitro kinase reaction, EphB3 immunoprecipitates were washed three times with lysis buffer and two times with kinase buffer (20 mM HEPES, pH 7.5; 1 mM DTT; 1 mM Na 3 VO 4 ; 10 mM MnCl 2 ). Kinase assay was performed in 40 μl of kinase buffer supplemented with 10 μg of the GST–JM substrate and 200 μM of ATP (Cell Signaling) for 30 min at 30°C. Reactions were stopped with loading buffer, boiled and samples analysed by western blotting. The tyrosine phosphorylation levels of GST–JM substrate were detected with phospho-tyrosine antibody pY100. Yeast two-hybrid screening A DNA fragment encoding the cytoplasmic portion of human EphB3 was subcloned into pGBKT7 (Clontech Laboratories) to yield a fusion protein with the Gal4 DNA-binding domain. This Gal4–EphB3 fusion protein was used as the bait for screening a human brain cDNA library (Clontech Laboratories) in pACT2 according to the manufacturer's instructions. Yeast transformation was performed in the strain AH109 with the polyethylene glycol-lithium acetate method, and positive clones were obtained by growing on selective media. DNA inserts from candidate clones were analysed by sequencing. RNA interference of RACK1 or PP2A Two target sequences for RACK1 and two for PP2A catalytic subunit-α small interfering RNA are listed in Supplementary Table S2 , respectively. Oligonucleotide with a scrambled sequence was used as a negative control. FG12 lentiviral vector was used to produce small double-stranded RNA (small interfering RNA) to inhibit target gene expression. Cell stimulation, immunoprecipitation and immunoblotting For EphB3 kinase activation, cells were stimulated with 2 μg ml −1 ephrin-B1–Fc, ephrin-B2–Fc or Fc control for 15 min at 37°C. For inhibition of EphB3 binding to endogenous ephrin-B1 or ephrin-B2, cells were treated for 3 h with 5 μg ml −1 EphB3–Fc or Fc control. In some experiments, H520/EphB3 stable cells were treated with CA or OA for indicated times before stimulation with ephrin-B1–Fc. Cells were lysed in RIPA buffer or 1% Triton X-100 buffer for western blot or immunoprecipitation, respectively. Samples were analysed by SDS–PAGE followed by immunoblotting with specific antibodies. Sequential coimmunoprecipitation assay Sequential coimmunoprecipitation was performed essentially according to the procedures described previously [46] . Briefly, HEK 293T cells were transfected with HA–EphB3, Flag–RACK1, Myc–PP2A and Akt. EphB3 lacking the HA-tag and Myc-tagged RACK1 were used as control for the first and second immunoprecipitation, respectively. At 24 h after transfection, the cells were lysed with lysis buffer (1% Triton X-100), sonicated briefly, and centrifuged. The supernatant was incubated with anti-HA antibody and protein A/G–agarose beads for 4 h at 4 °C. The beads were washed with lysis buffer three times, and the HA–EphB3 protein complex was eluted with 300 ml of lysis buffer containing 250 mM NaCl and HA peptide (Sigma-Aldrich) for 3 h at 4°C. Second immunoprecipitation was performed using anti-Flag antibody followed by elution with 3× Flag (Sigma-Aldrich) peptide in the same way. The second eluate was then subjected to the third immunoprecipitation with anti-Myc antibody or control IgG followed by the addition of protein A/G–agarose beads. Statistical analysis For parametric data sets, statistical significance was assessed by Student's t -test (analysis with SPSS software). How to cite this article: Li, G. et al . EphB3 suppresses non-small-cell lung cancer metastasis via a PP2A/RACK1/Akt signalling complex. Nat. Commun. 3:667 doi: 10.1038/ncomms1675 (2012).